Tuning the electron transport at single donors in zinc oxide with a scanning tunnelling microscope In devices like the single-electron transistor the detailed transport properties of a nanostructure can be measured by tuning its energy levels with a gate voltage. The scanning tunnelling microscope in contrast usually lacks such a gate electrode. Here we demonstrate tuning of the levels of a donor in a scanning tunnelling microscope without a third electrode. The potential and the position of the tip are used to locally control band bending. Conductance maps in this parameter space reveal Coulomb diamonds known from three-terminal data from single-electron transistors and provide information on charging transitions, binding energies and vibrational excitations. The analogy to single-electron transistor data suggests a new way of extracting these key quantities without making any assumptions about the unknown shape of the scanning tunnelling microscope tip. As the size of semiconductor devices decreases, individual dopants become decisive for the performance of devices [1] , [2] . Moreover, spin [3] or charge [4] states of single dopants have been proposed as key components of a solid-state quantum computer. The scanning tunnelling microscope (STM) has been used to characterize defect states of single dopants [2] and to manipulate their position and charge state [5] , [6] , [7] , [8] . There are predictions that double donors, which can deliver two electrons, may be particularly useful for addressing spin states in quantum computers [9] , [10] . In artificial atoms, as realized in a single-electron transistor (SET), it is possible to tune the energies of electronic states using a gate electrode. In contrast to single atoms on metal surfaces, whose ground state is determined by the impurity-substrate combination, transport experiments at different gate voltages can explore a wider parameter space. Signatures of single donors have been resolved and valuable information such as the electron-binding energy have been extracted [11] , [12] , [13] , [14] . Being a two-terminal device STM lacks a gate electrode for tuning the energy levels of nanostructures. To avoid this limitation, lithography has been used to fabricate a back gate [15] , [16] or source and drain contacts with the STM tip acting as a moveable gate [17] , [18] , [19] . Here we present an experimental approach to tune the levels of single quantum defects without a third electrode. It relies on the local band bending induced by the STM tip, which may be controlled by two independent parameters, the tip position and the sample voltage. Maps of the differential conductance in this parameter space closely resemble the Coulomb diamonds known from three-terminal experiments on SETs [20] and provide information on charge transitions, binding energies and vibrational excitations. We analyse double donors—most likely Zn interstitials [21] —close to the ZnO(0001) surface by measuring the differential conductance dI / dV versus lateral position x and sample voltage V , and show that a conventional two-terminal STM may be used to acquire SET-like data. Tip-induced band bending Nominally, undoped ZnO exhibits n -type conductivity, presumably due to intrinsic defects like Zn interstitials [21] , [22] . On our samples, we observed donor densities of ≈0.7…1.5 × 10 12 cm −2 . When the Au tip is brought close to an n -type ZnO crystal at zero bias voltage, the work function difference between the two materials causes the energy bands of ZnO to bend upwards. A positive (negative) voltage applied to the sample can increase (decrease) the band bending. Thus, the work function difference and the bias voltage result in a tip-induced band bending (TIBB). Its lateral extension depends on the tip radius of curvature and the tip-sample distance along with material parameters. Consequently, the applied voltage does not drop entirely inside the vacuum barrier but also inside the semiconductor and the chemical potential varies with depth and lateral distance to the STM tip. TIBB complicates the interpretation of dI / dV spectroscopy data because it shifts spectroscopic features. Moreover, it may move states across the Fermi energy of the semiconductor, thus changing their occupation and inducing additional spectral features. 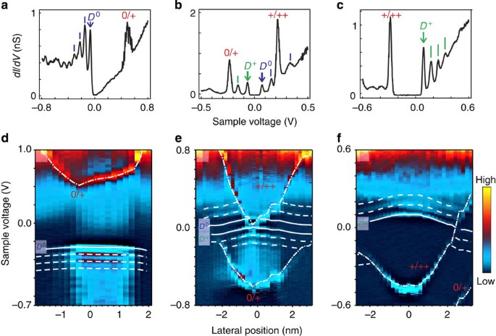Figure 1: Spectra of the differential conductance (dI/dV) of donors in ZnO. At zero bias, the donors are (a) neutral, (b) singly charged and (c) doubly charged.D0andD+indicate the levels of the donors, 0/+ and +/++ mark ionization peaks. At voltages below (above) 0/+ the donor is neutral (singly charged). +/++ marks transitions between the singly and the doubly charged states. Vertical bars indicate resolved vibrational features. Tunnelling parameters before disabling current feedback:I=3.0 nA,V=1.0, 0.5 and 0.6 V, respectively. Panelsd–fshow spatially resolved colour-codeddI/dV(x,V) maps from donors that are (d) neutral, (e) singly charged and (f) doubly charged at zero bias. Before disabling current feedback, the STM was operated atI=3 nA and sample voltages of 1.0, 0.8 and 0.6 V, respectively. The colour range corresponds to conductances of 0–1.2, −0.2–1.4 and 0–1.5 nS. Scans were performed along a line oriented 13° with respect to adirection. Simulation results are shown with lines. Dash dotted, solid and dashed lines indicate ionization lines (0/+ and +/++), defect levels (D0andD+) and vibrational satellites, respectively. While spectra like indwere observed from isolated donors,e,fwere typically found from closely spaced donors. In (d) the vibrational energyħω+≈70 meV is essentially independent of the tip-donor distance and similar values were measured above other isolated donors. Differential conductance spectra Figure 1 shows typical examples of differential conductance spectra from three classes of donors that correspond to different occupations with electrons at zero bias. The pronounced features can be attributed to donor states, charge transitions and vibronic excitations. The assignment of the observed signatures to specific processes and the identification of the charge state will become obvious below, when the lateral position x of the tip will be used as an additional parameter. The defect level of the donor of Fig. 1a is doubly occupied and the donor thus is neutral at zero bias [21] . The STM tip can extract electrons from the donor state resulting in a peak at a negative sample voltage (marked D 0 ). In addition, an equidistant sequence of vibronic excitations (vertical bars) is observed. The peak at positive sample bias (marked 0/+) corresponds to the voltage required to shift the donor state above the Fermi energy of the sample, which changes the charge of the donor from neutral to + e . Such ionization signatures in dI / dV spectra have also been observed on subsurface dopants in other semiconductors [6] , [23] , topological insulators [24] and molecular thin films [25] , as well as on adatoms on graphene [26] . The donor of Fig. 1b is singly occupied at zero bias. Thus, the STM tip can add or remove an electron at positive and negative voltages, respectively. Correspondingly, the ‘donor level’ appears twice in the spectrum as peaks D 0 and D + surrounding the Fermi energy E F . The splitting between these features is related to the Coulomb repulsion between two electrons in the donor level and will be discussed below in conjunction with the Coulomb blockade regime of the SET. In addition, two ionization peaks are observed (marked by 0/+ and +/++) that indicate the transitions from the singly charged to the neutral and doubly charged configurations, respectively. In Fig. 1c , the donor level is empty at zero bias. Thus, electrons can be added by the STM tip resulting in a peak (marked D + ) above E F along with vibronic transitions. A negative bias voltage can pull the defect level below E F of the sample resulting in a singly occupied state and a sharp peak in the dI / dV spectrum. Figure 1: Spectra of the differential conductance ( dI/dV ) of donors in ZnO. At zero bias, the donors are ( a ) neutral, ( b ) singly charged and ( c ) doubly charged. D 0 and D + indicate the levels of the donors, 0/+ and +/++ mark ionization peaks. At voltages below (above) 0/+ the donor is neutral (singly charged). +/++ marks transitions between the singly and the doubly charged states. Vertical bars indicate resolved vibrational features. Tunnelling parameters before disabling current feedback: I =3.0 nA, V =1.0, 0.5 and 0.6 V, respectively. Panels d – f show spatially resolved colour-coded dI/dV ( x,V ) maps from donors that are ( d ) neutral, ( e ) singly charged and ( f ) doubly charged at zero bias. Before disabling current feedback, the STM was operated at I =3 nA and sample voltages of 1.0, 0.8 and 0.6 V, respectively. The colour range corresponds to conductances of 0–1.2, −0.2–1.4 and 0–1.5 nS. Scans were performed along a line oriented 13° with respect to a direction. Simulation results are shown with lines. Dash dotted, solid and dashed lines indicate ionization lines (0/+ and +/++), defect levels ( D 0 and D + ) and vibrational satellites, respectively. While spectra like in d were observed from isolated donors, e , f were typically found from closely spaced donors. In ( d ) the vibrational energy ħω + ≈70 meV is essentially independent of the tip-donor distance and similar values were measured above other isolated donors. Full size image Differential conductance maps To further confirm the peak assignment, we measured series of dI / dV spectra at densely spaced positions along straight lines crossing the buried donors. These data are shown as two-dimensional colour-coded maps in Fig. 1d–f . The maps display one ( Fig. 1d ) or two ( Fig. 1e,f ) conductance maxima that appear as approximate parabolae (dash dotted lines). These parabolae are due to the ionization peaks introduced in Fig. 1a–c and are labelled accordingly. The variation of the ionization peaks with lateral position is due to the change of the TIBB at the position of the donor. To pull an occupied level above E F , a small positive voltage is required if the donor is right below the tip ( D 0 in Fig. 1d , and D + in Fig. 1e). This voltage is increased at larger separations, which gives rise to the parabolae observed at V >0 in Fig. 1d,e . The parabolae at negative sample bias are due to empty levels that are pushed below E F ( D 0 in Fig. 1e and D + in Fig. 1f). This requires the contact potential, which is maximal below the tip, be compensated. The voltage | V | for ionization therefore is largest for a donor below the tip apex [27] . The variation of the donor levels D 0 and D + and the vibrational excitations with lateral position reflects the TIBB in the semiconductor. Data analysis In previous modelling of STM measurements on subsurface dopants, the Poisson equation was solved to determine the TIBB [6] , [23] . This involves a number of parameters. While some of them, for example, the band gap and the dielectric constant, may be taken from literature, others such as the tip-sample separation, the radius of curvature of the tip and its shank angle are a priori unknown and have to be adjusted to match the experimental data. In our approach, the donor is modelled by a single orbital with an energy ε d (defined with respect to the local chemical potential μ c ) and a Coulomb repulsion U in the case of double occupancy. The total energies E n for occupation numbers n =0, 1 and 2 are and correspond to the doubly charged, singly charged and neutral configurations, respectively. For sample voltages V below the inversion threshold and above flat band conditions, no charge accumulation occurs at the surface and the TIBB may be assumed to vary linearly with the bias voltage [28] . This leaves the factor β ( x ) and the flat band voltage V F as parameters to be extracted from the experimental data. β ( x ) resembles the shape of the TIBB as a function of lateral distance x and in a fixed depth inside the semiconductor. To calculate the illustrative examples in Fig. 2 and Supplementary Fig. 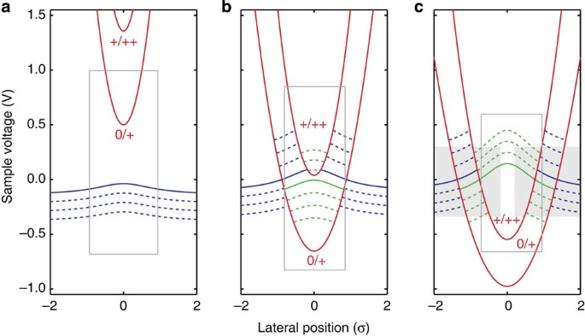Figure 2: Calculated energy diagrams. Calculated energy diagrams over a wide range of voltages and distances for a symmetric model tip where β(x) is assumed to be a squared Lorentzian of widthσ. Parameters ina–cwere adjusted to approximate the data shown inFig. 1d–f, respectively, which correspond to the areas marked by grey rectangles. Red curves represent the ionization lines. Blue and green solid lines are the donor levels ofD0andD+, dashed lines display the vibrational satellites. The shaded area incexhibits a striking similarity to Coulomb blockade diamonds. S1 , we used an analytical expression for β that models the lateral variation of the TIBB at a given depth by a squared Lorentzian of width σ : Figure 2: Calculated energy diagrams. Calculated energy diagrams over a wide range of voltages and distances for a symmetric model tip where β( x ) is assumed to be a squared Lorentzian of width σ . Parameters in a – c were adjusted to approximate the data shown in Fig. 1d–f , respectively, which correspond to the areas marked by grey rectangles. Red curves represent the ionization lines. Blue and green solid lines are the donor levels of D 0 and D + , dashed lines display the vibrational satellites. The shaded area in c exhibits a striking similarity to Coulomb blockade diamonds. Full size image The ionization voltages V +/++ and V 0/+ fulfil the conditions E 0 = E 1 and E 1 = E 2 , respectively, and separate ground states with different occupation numbers. They are given by and Since these conditions can always be met, two ionization parabolae (red curves in Fig. 2 ) are present in every dI / dV map. The data furthermore provide an opportunity to determine vibrational energies ħω n of a donor in different charge states. For instance, in Fig. 1d , an electron is extracted from a neutral donor at V< 0. The vibronic features therefore reflect the vibrational energy of a singly charged donor [29] , [30] . In contrast, Fig. 1e shows the vibrations of a donor in its neutral and doubly charged states for V >0 and V< 0, respectively. In our model, we allow the vibration energies ħω n to depend on the occupation number n and hence on the charge of the donor. For positive V direct tunnelling into the donor state increases n by one ( n → n +1) and m vibronic modes of energy ħω n +1 may be excited. This excitation requires an energy eV > = E n +1 − E n + mħω n +1 . Electron extraction at negative V decreases the occupation ( n → n −1) while exciting m vibrations in charge state n −1. The required energy is − eV < = E n −1 − E n + mħω n −1 . From the above equations we derive the following: For the elastic transitions ( m =0), we simplify the terminology of the above expressions to and . These expressions define the bias voltages of all spectroscopic features depicted in Fig. 2 , namely, ionization lines V +/++ and V 0/+ (red), donor levels and (solid blue and green) and vibrational satellites (dashed blue and green). We have applied the model to different kinds of donors ( Supplementary Note 1 and Supplementary Table S1 ). An analysis of a number of donors reveals that the vibrational energy depends on the charge state ( Supplementary Note 2 and Supplementary Fig. S2 ). The extracted binding energies, Coulomb repulsions and vibrational energies in different charge states are displayed in Table 1 and the Supplementary Table S2 . Table 1 Microscopic parameters (in meV) obtained from five donors . Full size table A simplified presentation of the spectroscopic features of Fig. 1 is obtained by performing calculations for a symmetric tip and neglecting the local environment of the donors. Figure 2a and b correspond to the cases of neutral and singly charged donors of Fig. 1d and e , respectively. Figure 2c displays the most interesting case. In the shaded area, the intersections of the donor levels D 0 and D + and the ionization lines 0/+ and +/++ are the four corners of a diamond-shaped area in the x − V plane where the differential conductance vanishes because of Coulomb blockade. In a SET ( Fig. 3a ), the energies of states and their occupations can be controlled by a gate voltage V G while the current is driven between source and drain contacts using a voltage V SD . The differential conductance of a SET may be schematically described by the diagram in Fig. 3c . Lines with negative (positive) slope indicate conductance peaks that occur when the donor levels are in resonance with the Fermi level of the source (drain) contact. n =0, 1 or 2 indicates the occupation numbers of the nanostructure at V SD =0. In the shaded areas Coulomb blockade occurs. The dI / dV ( x , V ) map of a donor under a STM tip ( Fig. 3d ) is closely related. While the sample voltage V corresponds to V SD in a SET, the tip position x plays the role of V G . In the experiments it was difficult to obtain a dI / dV map with all n =0, 1, 2 regions from a single donor. Therefore, Fig. 3e and g show data from two different donors, which exhibit occupations n =0, 1 and n =1, 2, respectively. The schematics in Fig. 3f,h label the main spectral features. 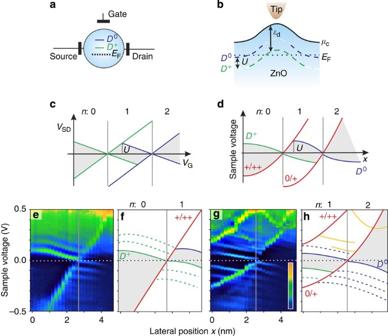Figure 3: Analogy between a donor in a SET and underneath a STM tip. (a) Schematics of a SET. Current is passed between the source and drain contacts via two localized levelsD0andD+, which can be shifted by applied voltage to the insulated gate contact. In the indicated case the donor is doubly charged. (b) Schematic diagram of local band bending in a semiconductor underneath a STM tip.μc, local chemical potential, εd, binding energy of the first electron in the donor level. The levelsD0andD+are marked by blue and green dashed lines when accessible by single-particle transitions and are coloured white otherwise. (c) Schematic two-dimensional map of conductance maxima of the SET versus source-drain voltageVSDand gate voltageVG.nis the occupation number. Depending onVG, the number of electrons in the donor changes fromn=0 over 1 to 2. (d) Variation of the donor levelsD0andD+(blue and green solid lines) and the ionization lines (0/+) and (+/++) (red lines) with distancexfrom the tip apex and sample voltageV. Incanddvertical dotted lines indicate the Coulomb energyU. (e,g)dI/dV(x,V) maps recorded along straight lines crossing buried donors. Before disabling current feedback, the STM was operated at 0.5 V, 3 nA. The colour bar represent 0–2 nS in both maps. Panelsfandhsketch the main conductance maxima fromeandg. Dotted lines indicate vibrational satellites. Yellow lines inhmark features that are attributed to nearby defects. Inc,d,fandh, shaded areas show Coulomb blockade. Figure 3: Analogy between a donor in a SET and underneath a STM tip. ( a ) Schematics of a SET. Current is passed between the source and drain contacts via two localized levels D 0 and D + , which can be shifted by applied voltage to the insulated gate contact. In the indicated case the donor is doubly charged. ( b ) Schematic diagram of local band bending in a semiconductor underneath a STM tip. μ c , local chemical potential, ε d , binding energy of the first electron in the donor level. The levels D 0 and D + are marked by blue and green dashed lines when accessible by single-particle transitions and are coloured white otherwise. ( c ) Schematic two-dimensional map of conductance maxima of the SET versus source-drain voltage V SD and gate voltage V G . n is the occupation number. Depending on V G , the number of electrons in the donor changes from n =0 over 1 to 2. ( d ) Variation of the donor levels D 0 and D + (blue and green solid lines) and the ionization lines (0/+) and (+/++) (red lines) with distance x from the tip apex and sample voltage V . In c and d vertical dotted lines indicate the Coulomb energy U . ( e , g ) dI/dV ( x,V ) maps recorded along straight lines crossing buried donors. Before disabling current feedback, the STM was operated at 0.5 V, 3 nA. The colour bar represent 0–2 nS in both maps. Panels f and h sketch the main conductance maxima from e and g . Dotted lines indicate vibrational satellites. Yellow lines in h mark features that are attributed to nearby defects. In c , d , f and h , shaded areas show Coulomb blockade. Full size image The analogy between STM and SET suggests a route to determine the Coulomb repulsion U ( Fig. 3c,d ). It may be read off directly from the intersections of the conductance features D 0 and (+/++) (dashed vertical lines). At these voltages, ε d + U and ε d are aligned with the Fermi levels of the tip and of ZnO, respectively. In the same way, D + and (0/+) intersect at − U . In summary, we used a conventional two-terminal STM to perform measurements that are comparable to those in a three-terminal SET. dI / dV ( x , V ) maps reveal that donors may be classified according to their charge states at zero bias. The donors display Coulomb blockade and charge-state-dependent vibrational energies. They are analysed by a new model that is inspired by the analogy to a SET. The method may also be useful for other nanostructures buried in a semiconductor matrix. It may become possible to observe the influence of their charge state on the Kondo effect, metal–insulator transitions, or Franck–Condon blockade, similar to observations made from SET [20] , [31] but on a much smaller length scale. Experimental details All experiments were performed with a home-built STM operated at 5 K in ultra-high vacuum. Wurtzite ZnO(0001) single crystals were cleaned by Ar + bombardment and high temperature annealing. Imaging was performed at constant current with Au tips and the bias voltage was applied to the sample. Ex situ cut tips were gently brought into mechanical contact to the ZnO surface and retracted again. This procedure typically lead to the deposition of a Au cluster and often improved the sharpness of the tips. Spectra of dI / dV were measured with a lock-in amplifier using a sinusoidal modulation of the bias with amplitudes of 10−15 mV rms . Analytical model For quantitative analysis of the energies of the spectral features, the applied sample voltage must be converted into a chemical potential at the position of the donor. We thus define a scaling factor β ( x ) to describe the change of the chemical potential μ c ( x , V )= β ( x ) e ( V − V F ) due to the voltage V . V F is the flat band voltage and β ( x ) is a tip-specific function that resembles the shape of the TIBB as a function of lateral distance x . The donor is described by a single level with energy ε d with respect to the local chemical potential and an on-site Coulomb repulsion U between two electrons in the localized state. β ( x ), V F , ε d and U are then determined by fitting the calculated energies to the experimental peak positions. Usually, retrieving such quantitative information from experiments is complicated by the unknown geometry of the tunnelling junction, which affects the TIBB. The present approach circumvents this problem as the tip-shape influences β ( x ), which is extracted from the experimental data. We also compared the result with calculation using Poisson equations ( Supplementary Fig. 3 and Supplementary Note 3 ). How to cite this article: Zheng, H. et al. Tuning the electron transport at single donors in zinc oxide with a scanning tunnelling microscope. Nat. Commun. 4:2992 doi: 10.1038/ncomms3992 (2014).